Tie-mediated signal from apoptotic cells protects stem cells inDrosophila melanogaster Many types of normal and cancer stem cells are resistant to killing by genotoxins, but the mechanism for this resistance is poorly understood. Here we show that adult stem cells in Drosophila melanogaster germline and midgut are resistant to ionizing radiation (IR) or chemically induced apoptosis and dissect the mechanism for this protection. We find that upon IR the receptor tyrosine kinase Tie/Tie-2 is activated, leading to the upregulation of microRNA bantam that represses FOXO -mediated transcription of pro-apoptotic Smac/DIABLO orthologue, Hid in germline stem cells. Knockdown of the IR-induced putative Tie ligand, Pvf1 , a functional homologue of human Angiopoietin , in differentiating daughter cells renders germline stem cells sensitive to IR, suggesting that the dying daughters send a survival signal to protect their stem cells for future repopulation of the tissue. If conserved in cancer stem cells, this mechanism may provide therapeutic options for the eradication of cancer. A form of programmed cell death, apoptosis, is characterized as controlled, caspase-induced degradation of cellular compartments to terminate the activity of the cell. Apoptosis plays a vital role in various processes including normal cell turnover, proper development and function of the immune system and embryonic development [1] , [2] . Apoptosis is also induced by upstream signals, such as DNA double-strand breaks (DSB), to destruct severely damaged cells [3] , [4] . DSB activate ATM checkpoint kinase and Chk2 kinase-dependent p53 phosphorylation and induction of repair genes. However, if DSB are irreparable, p53 activation will result in pro-apoptotic gene expression and cell death [5] , [6] , [7] . However, aggressive cancers contain cells that show inability to undergo apoptosis in response to stimuli that trigger apoptosis in sensitive cells [8] , [9] . This feature is responsible for the resistance to anticancer therapies, as well as the relapse of tumours after treatment, yet the molecular mechanism of this resistance is poorly understood. As the cell type that constantly regenerates and gives rise to differentiated cell types in a tissue, stem cells share high similarities with cancer stem cells, including unlimited regenerative capacity and resistance to genotoxic agents [10] . Adult stem cells in model organisms such as Drosophila melanogaster , have been utilized to study stem cell biology and for conducting drug screens, thanks to their intrinsic niche, which provides authentic in vivo microenvironment [11] , [12] , [13] . In this study, we show that Drosophila adult stem cells are resistant to radiation/chemical-induced apoptosis and dissect the mechanism for this protection. We show that a previously reported cell survival gene with a human homologue, pineapple eye (pie) , acts in both stem cells and in differentiating cells to repress the transcription factor FOXO . Elevated FOXO levels in pie mutants lead to apoptosis in differentiating cells, but not in stem cells, indicating the presence of an additional anti-apoptotic mechanism(s) in the latter. We show that this mechanism requires Tie , encoding a homologue of human receptor tyrosine kinase Tie-2 , and its target, bantam , encoding a microRNA. The downstream effector of FOXO , Tie and ban , we show is Hid , encoding a Smac/DIABLO orthologue. Knocking down the ligand Pvf1/PDGF/VEGF/Ang in differentiating daughter cells made stem cells more sensitive to radiation-induced apoptosis, suggesting that Pvf1 from the apoptotic differentiating daughter cells protects stem cells. Drosophila stem cells resist IR/maytansinol caused apoptosis External stress, such as ionizing radiation (IR), induces DNA damage and apoptosis in Drosophila [14] . In the apical tip of the germarium of the Drosophila ovary, two to three germline stem cells (GSCs), marked by spherical spectrosomes (SS), are in direct contact with the somatic niche composed of terminal filaments and cap cells ( Fig. 1a ). The GSC divides asymmetrically along the anterior–posterior axis from the niche, producing a GSC and a transit-amplifying (TA) daughter cystoblast (CB). The CB further divides to form a 2–16 cell cyst containing interconnected cells ( Fig. 1a ) [15] . We found that the multi-cell cysts, marked by branched fusomes, were eliminated within 3 days after exposure to 50 Gy of γ-rays ( Fig. 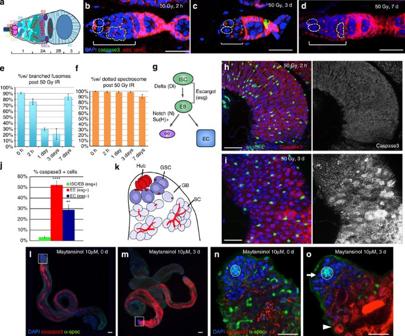Figure 1: Ionizing radiation and maytansinol caused cell death in differentiated cells but not in stem cells. (a) Diagram showing the germarium ofDrosophilaovary. GSCs (GSC, pink) indicated by anterior spectrosomes (SS, red) are located at the anterior end of the germarium adjacent to the niche cap cells (CpC, light green). Escort stem cell (ESC, lavender), differentiated CB (blue), germ cell cyst marked by the presence of branched fusomes (BS, red), somatic stem cells (SSCs, violet), follicle cells (FC, light blue). (b–d) w- germarium representative of three experiments* from 2 h, 3 days and 7 days post 50 Gy gamma-irradiation (IR). White dashed circles mark the GSCs. Brackets indicate stages 1 and 2A. Adducin and LaminC (red); cleaved caspase 3 (green); DAPI (4,6-diamidino-2-phenylindole; blue). Scale bar, 20 μm. (e) Mean percentage of germaria with branched fusomes in w-females at 0 h (n=398), 2 h (n=173), 1 day (n=203), 3 days (n=148) and 7 days (n=171) post 50 Gy IR. (f) Mean percentage of germaria with dotted spectrosome adjacent to the niche at 0 h, 2 h, 1 day, 3 days and 7 days post 50 Gy IR. Error bars, s.d. (g) Diagram ofDrosophilaISC and the differentiated progenies. EB (green), EC (blue), ee cells (purple). (h–i) Posterior midgut of esgGal4; UAS-GFP adults 2 h and 3 days post 50 Gy IR. Scale bar, 75 μm. (j) Mean percentage of cleaved caspase3+ cells in ISC/EB (n=197), ee (n=251), and EC cell types (n=818) respectively. Error bar, s.e.m. (k) Schematic diagram of theDrosophilamale GSC niche. SC, spermatocytes. Dotted and branched fusomes are indicated in red in GSCs and differentiated cells. (l–m)Drosophilatestis before and after 10 μM maytansinol feeding. Cleaved caspase3 (red). Scale bar, 75 μm. (n-o) Male GSC niche before and after 3 days 10 μM maytansinol treatments. Arrow points at GSC adjacent to the niche; arrowhead points at differentiated germline cell with cleaved caspase3 expression. Scale bar, 20 μm. *All figures are representative of at least three experiments unless stated otherwise. 1b,c,e ; Supplementary Table 1 ), resulting in a significantly diminished region 1-2A in germarium (bracket length). Most of the remaining cells, including the 2-3 closely attached to the somatic niche, are labelled with SSs, indicating the GSC identity ( Fig. 1c , dashed circles, f; Supplementary Table 1 ). We conclude that irradiation results in the loss of differentiating cyst cells but not GSCs. Importantly, 7 days post-IR treatment, the multi-cell cysts were observed again in the germaria ( Fig. 1d-e ), indicating that the irradiated GSCs are able to repopulate the tissue. Figure 1: Ionizing radiation and maytansinol caused cell death in differentiated cells but not in stem cells. ( a ) Diagram showing the germarium of Drosophila ovary. GSCs (GSC, pink) indicated by anterior spectrosomes (SS, red) are located at the anterior end of the germarium adjacent to the niche cap cells (CpC, light green). Escort stem cell (ESC, lavender), differentiated CB (blue), germ cell cyst marked by the presence of branched fusomes (BS, red), somatic stem cells (SSCs, violet), follicle cells (FC, light blue). ( b – d ) w- germarium representative of three experiments* from 2 h, 3 days and 7 days post 50 Gy gamma-irradiation (IR). White dashed circles mark the GSCs. Brackets indicate stages 1 and 2A. Adducin and LaminC (red); cleaved caspase 3 (green); DAPI (4,6-diamidino-2-phenylindole; blue). Scale bar, 20 μm. (e) Mean percentage of germaria with branched fusomes in w - females at 0 h ( n =398), 2 h ( n =173), 1 day ( n =203), 3 days ( n =148) and 7 days ( n =171) post 50 Gy IR. ( f ) Mean percentage of germaria with dotted spectrosome adjacent to the niche at 0 h, 2 h, 1 day, 3 days and 7 days post 50 Gy IR. Error bars, s.d. ( g ) Diagram of Drosophila ISC and the differentiated progenies. EB (green), EC (blue), ee cells (purple). ( h – i ) Posterior midgut of esgGal4; UAS-GFP adults 2 h and 3 days post 50 Gy IR. Scale bar, 75 μm. ( j ) Mean percentage of cleaved caspase3+ cells in ISC/EB ( n =197), ee ( n =251), and EC cell types ( n =818) respectively. Error bar, s.e.m. ( k ) Schematic diagram of the Drosophila male GSC niche. SC, spermatocytes. Dotted and branched fusomes are indicated in red in GSCs and differentiated cells. ( l – m ) Drosophila testis before and after 10 μM maytansinol feeding. Cleaved caspase3 (red). Scale bar, 75 μm. ( n-o ) Male GSC niche before and after 3 days 10 μM maytansinol treatments. Arrow points at GSC adjacent to the niche; arrowhead points at differentiated germline cell with cleaved caspase3 expression. Scale bar, 20 μm. *All figures are representative of at least three experiments unless stated otherwise. Full size image Another well-studied adult stem cell model is the intestinal stem cell (ISC) residing in Drosophila posterior midgut. The Drosophila midgut is composed of a simple columnar epithelium surrounded by visceral muscle. This simply structured organ consists of the following cell types: polyploid enterocytes (ECs); small diploid enteroendocrine cells (ee); and the common progenitors for these cells, the ISCs and their diploid daughter cells, enteroblasts (EBs). After an asymmetric division, an ISC renews itself while giving rise to a new EB cell, which later will differentiate into either ee or EC lineage ( Fig. 1g ) [16] , [17] , [18] . ISCs can be identified by their expression of the Notch ligand Delta (Dl) and the transcription factor escargot (esg ). Three days after exposure to 50 Gy of γ-rays, a marked increase in cleaved caspase 3 signal was observed in most of the midguts, suggesting induction of apoptosis ( Fig. 1h-j ). However, while a large proportion of ee and EC cells are apoptotic, only few esg+ cells (ISCs or EBs) displayed activated caspase3 signal ( Fig. 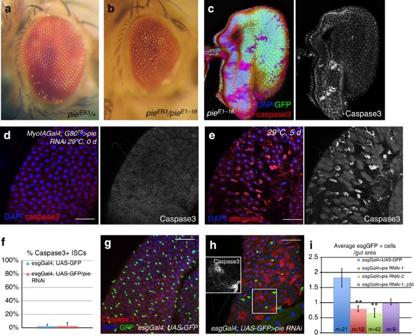Figure 2:pieis required for cell survival of somatic but not stem cells. (a)pieEB3/+ adults display normal compound eyes (anterior to the right). (b)pieEB3/ pieE1-16transheterozygous eyes are rough and irregular with variable facet size. (c) Third instar eye disc displays cleaved caspase3 inpieE1-16clones (GFP−). (d–e) Posterior midguts ofMyoIAGal4; tubGal80ts, UAS-GFP/pie RNAianimals 0 and 5 days after shifting to 29 °C. (f) Mean cleaved caspase 3 positive ISCs inesgGal4; UAS-GFPcontrol (g) (n=165) andesgGal4; UAS-GFP/pie RNAi(H) midguts (n=97). (g) Posterior midgut of controlesgGal4; UAS-GFPanimal. (h) Posterior midgut ofesgGal4; UAS-GFP/pie RNAianimal. Insets show absence of caspase3 (white) activity in ISCs. Scale bar, 75 μm. (i) Mean esgGFP+ cells normalized to gut area. Sample size specified in the graph. Error, s.d. 1j , Supplementary Table 2 ), indicating that this stem cell type is also resistant to apoptosis-induced by γ-rays. Further, positively marked Mosaic Analysis with a Repressible Cell Marker (MARCM) clones show that the post-IR ISCs are capable of generating multi-cell clones containing all cell lineages by day 6 ( Supplementary Fig. 1 ), demonstrating the repopulation capacity of the ISC post-irradiation. However, the clones generated from the IR-treated ISCs are of significantly smaller size compared with those from untreated ISCs ( Supplementary Fig. 1c ), suggesting a brief quiescent period due to irradiation, after which the stem cells resume self-renewing division and repopulate the tissue. At the apex of a Drosophila testis, post-mitotic somatic hub cells comprise a key component of the male GSC niche, supporting 10 to 12 GSCs ( Fig. 1k ). As in the female germline, daughters of male GSCs, known as gonialblasts (GBs), go through synchronous incomplete divisions to generate 16-cell cysts marked by highly branched fusomes [13] , [19] . Similar to ISCs and to female GSCs, testes exposed to 50 Gy of γ-rays also show a rapid loss of spermatocyte cysts while the GSCs remain in the stem cell niche ( Supplementary Fig. 2 ). IR (50 Gy) would also be sufficient to induce robust apoptosis in the Drosophila embryo and in diploid cells of the larvae [20] , [21] . We conclude that GSCs in the ovaries and the testes, and ISCs in the midguts are resistant to IR-induced apoptosis compared with their differentiating progenies. Radiation and chemotherapy are widely applied in treatments against cancers based on their ability to induce apoptosis. An anticancer chemical, maytansinol, a microtubule depolymerizing agent currently in clinical trials (for example, NCT01470456, www.clinicaltrials.gov ), has been reported to cause significant apoptosis in Drosophila and growth inhibition in human cancer cells [21] . Testes from adult flies fed with water containing 10 μ M maytansinol for 3 days showed marked apoptosis as indicated by increased cleaved caspase 3 ( Fig. 1l–m ). However, when the GSC niche was examined, no caspase 3 activity was observed in the stem cells ( Fig. 1n-o , arrow), despite the high caspase 3 expression induced in the differentiated cells (arrowhead). 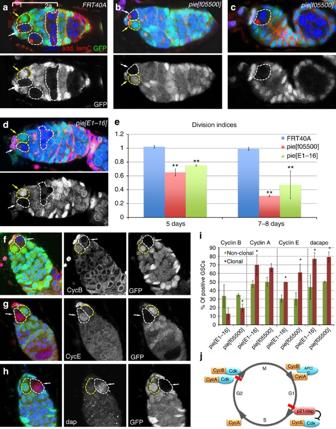Figure 3:pieis required for female GSC division. (a) Germarium ofhsFlp; Ubi-GFP FRT40A/FRT40Afemales, 8 days after heat shock. (b–c) Germaria ofhsFlp; Ubi-GFP FRT40A/ pief05500FRT40Afemales, 8 and 9 days after heat shock. (d) Germarium ofhsFlp; Ubi-GFP FRT40A/ pieE1-16FRT40Afemales, 8 days after heat shock. White arrow, clonal GSC; yellow arrow, non-clonal sister GSC; white dashed circle, progenies produced by clonal GSC within stage 1-2A. (e) Means of division indices ofFRT40A,pief05500andpieE1-16GSCs are calculated from samples collected, respectively, at 5 and 7-8 days after heat shock induction. Sample size specified inSupplementary Table 6. Error, s.d. In ovaries 8 days after heat shock induction,pief05500clonal GSCs (white dashed circles and arrows) display repressed expression of Cyclin B (f), elevated expression of Cyclin E (g) and dacapo (h), compared with non-clonal sister GSCs (yellow dashed circles). (i) Means of frequencies ofpiemutant (pief05500andpieE1-16) GSCs positive for each cell cycle marker compared with those of non-clonal sister GSCs. Sample size specified inSupplementary Table 7. Error, s.d. (j) Diagram of cell cycle phases and corresponding markers. In an ongoing screen for molecules capable of inducing apoptosis in adult stem cells, using NCI Diversity Set IV compound library, we observed that many other pro-apoptotic molecules also failed to induce apoptosis in male GSCs, even at high concentration ( Supplementary Table 3 ). These data, together with the above observation in irradiated tissues, demonstrates the special capacity of adult stem cells to resist damage-induced apoptosis. Inhibitor of apoptosis proteins (IAPs) inhibit caspases and function as the key inhibitors of apoptosis; DIAP1 is the major Drosophila homologue [3] . To test if the cell death can be induced genetically in the stem cells, we induced DIAP1 mutant clones in the female germline, and examined if the clonal stem cells can survive. As early as 3 days after clone induction, no mutant clones were observed in the stem cell niche, while the wild-type control clones were recovered in 15% of the germaria examined ( Supplementary Fig. 3 ), suggesting an acute loss of stem cells due to the removal of the essential protector, DIAP1 . These data suggest that while adult stem cells are capable of undergoing caspase cleavage and apoptosis, they normally utilize protection mechanism(s) against it. Pie as a survival factor in differentiated but not stem cells A previous screen for essential factors in stem cell self-renewal identified a cell survival factor, pie [22] . As the Drosophila homologue of human G2E3 ubiquitin ligase, pie was originally reported to be required for cell survival in the developing Drosophila eyes [23] , [24] . Consistent with the published reports, we observed marked rough eye phenotypes in the adult survivors transheterozygous for a null allele pie E1-16 and a hypomorphic allele pie EB3 ( Fig. 2a-b ). In larval eye discs, apoptosis marker cleaved caspase3 was detected in pie mutant clones ( Fig. 2c , green fluorescent protein (GFP−)), but not in wild-type cells (GFP+), indicating induced apoptosis in mutant cells. Figure 2: pie is required for cell survival of somatic but not stem cells. ( a ) pie EB3 /+ adults display normal compound eyes (anterior to the right). ( b ) pie EB3 / pie E1-16 transheterozygous eyes are rough and irregular with variable facet size. ( c ) Third instar eye disc displays cleaved caspase3 in pie E1-16 clones (GFP−). ( d – e ) Posterior midguts of MyoIAGal4; tubGal80ts, UAS-GFP/pie RNAi animals 0 and 5 days after shifting to 29 °C. ( f ) Mean cleaved caspase 3 positive ISCs in esgGal4; UAS-GFP control ( g ) ( n =165) and esgGal4; UAS-GFP/pie RNAi (H) midguts ( n =97). ( g ) Posterior midgut of control esgGal4; UAS-GFP animal. ( h ) Posterior midgut of esgGal4; UAS-GFP/pie RNAi animal. Insets show absence of caspase3 (white) activity in ISCs. Scale bar, 75 μm. ( i ) Mean esgGFP+ cells normalized to gut area. Sample size specified in the graph. Error, s.d. Full size image We used MyoIAGal4, an enterocyte-specific driver, to knockdown pie by RNAi in the ECs of the midgut. As in the case of the eye tissue, cleaved caspase 3 staining was strongly elevated in the EC ( Fig. 2d-e ), indicating that reduced pie resulted in apoptosis in the differentiated gut cells. In contrast, knocking down pie in ISCs using an esgGal4 driver did not result in elevated caspase3 signal ( Fig. 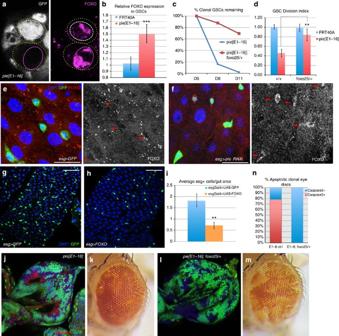Figure 4:pieregulates GSC self-renewal throughFOXOlevel. (a) Eight to eleven days after clone induction,pieE1-16clonal GSC nucleus (GFP−, magenta dashed circle) display higher expression ofFOXOcompared with sister non-clonal GSC nucleus (GFP+, white dashed circle). Yellow dashed circles mark the whole GSCs. (b) Quantification of relativeFOXOexpression levels (clonal versus non-clonal) inpieE1-16GSCs andFRT40Acontrols. Sample sizes refer toSupplementary Table 8. Error, s.d. (c) Heterozygous mutantfoxo25/+ rescues the rapid loss ofpieE1-16GSCs. Each data point represents mean of three independent experiments. (d) Heterozygous mutantfoxo25/+ rescues division defects ofpieE1-16GSCs. Sample sizes refer toSupplementary Table 9. Error, s.d. (e) ISCs from wild-type midguts have undetectableFOXOlevel while pie RNAi knockdown ISCs stained positive for anti-FOXO antibody (f, red arrows). Scale bar, 20 μm. (g–h) Posterior midguts ofesgGal4, UAS-GFP>UAS-GFP(g) andesgGal4, UAS-GFP>UAS-FOXO(h) adults. Scale bar, 75 μm (i) Means of esgGFP+ cell numbers normalized to quantified gut area (esgGal4>GFP:n=15; esgGal4>FOXO:n=11). Error, s.d. (j) Eye disc from 3rdinstar larva withpieE1-16clones (GFP-) and (k) fly eye developed into adulthood. (l) Eye disc from 3rdinstar larva withpieE1-16; foxo25/+ clones (GFP−) and (m) fly eye developed into adulthood. (n) Quantification of eye discs with or without apoptotic clones inpieE1-16(n=25) andpieE1-16; foxo25/+ (n=22) larvae. 2f,h ; Supplementary Table 4 ). This is in agreement with previous observations that loss of pie in GSCs does not induce apoptosis [22] . However, esgGal4 driven pie RNAi expression did lead to a significant reduction of the esg+ cells, which was not rescued by the co-expression of the caspase inhibitor p35 ( Fig. 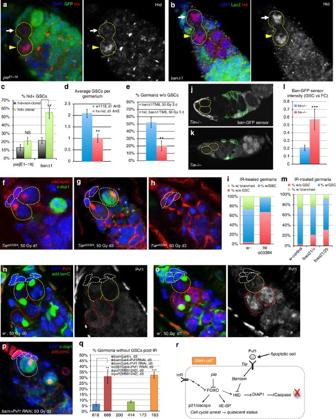Figure 5:Pvf1from dying daughters activatesTieto protect stem cell from apoptosis through bantam-regulatedhidlevel. (a)hsFlp;Ubi-GFP FRT40A/pieE1-16FRT40Aand (b)hsFlp;; armLacZ FRT80B/ banΔ1 FRT80Bgermarium 8 days after heat shock. Yellow dashed line circles clonal GSC and its CB daughter. White arrows: GSCs; yellow arrowheads: cystoblasts. (c) Means of percentage of hid+ clonal GSCs and non-clonal neighbor GSCs ofpieE1-16(n=97) andbanΔ1(n=57) background. NS: not significant. (d) Mean GSC numbers per germarium ofw1118(n=44) andhs-Hid(n=38) females, 1 day after heat shock treatment. (e) Means of percentage of germaria without GSCs inbanΔ1/TM6(n=160) andhidl(3)05014,banΔ1/TM6(n=191) females 3 days after IR.tiee03394mutant germarium one day (f) and 3 days (g–h) post 50 Gy IR treatment. White dashed circles mark the somatic cap cells; yellow dashed circles indicate GSCs labelled by dotted spectrosomes (absent inh); cleaved dcp-1 (green) indicates apoptotic cells. (i) Percentages of germaria with branched fusomes (green), with only GSCs (blue), and absent of any GSCs (red) are shown for w- (n=204) andtiee03394mutant (n=270) 3 days post 50 Gy IR. (j–l) ban-GFP sensor activity quantified as intensity in GSCs (yellow dashed circles) normalized against follicle cells (green dashed outlined), intieDf/+ (n=12) andtieDf/Df(n=8) females. (m) Percentages of germaria with branched fusomes (green), with only GSCs (blue), and absent of any GSCs (red) are shown for w- (n=61),foxo21/+ (n=105) andfoxo21/foxo25mutants (n=287) 3 days post IR. (n)w1118germarium pre and (o) 1 day post 50 Gy IR. White dashed circles mark the cap cells; yellow dashed circles indicate GSCs labelled by dotted spectrosomes facing the niche; red dashed circles mark differentiated cystoblasts. Note Pvf1 expression is markedly elevated in the cystoblasts post IR (o). (p) Germarium ofbamGal4/Pvf1 RNAiadults 3 days post 50 Gy IR. Apoptotic GSC shows cleaved dcp-1 activity (green). (q) Mean percentages of germaria absent of GSCs from various genotypes are shown. Sample size specified at the bottom. Notepvf1MB0124250 Gy d3is highly significant (***P≤0.001) compared with eitherbamGal4/+,50 Gy d3orpvf1MB0124250 Gy d0. (r) Proposed mechanism of how female GSCs are protected against apoptosis through joint efforts from multiple signalling pathways. Error, s.d. 2g-i ; Supplementary Table 5 ). Although widely used as an ISC marker, esg is expressed in both ISCs and their immediate daughter cell EBs. By examining the expression of EB marker Suppressor-of-Hairless ( Su(H) ), we identified that the majority of the remaining esg+ cells in pie knockdown midguts posses EB identity, while in wild type only half of the total esg+ cells are EBs ( Supplementary Fig. 4 ). Furthermore, knocking down pie specifically in EBs using Su(H)Gal4 driver did not affect neighbouring ISC numbers ( Supplementary Fig. 5 ), excluding the possibility that pie non-autonomously regulates ISCs through EBs. These data conclusively indicate that pie is specifically required for ISC maintenance, but not through apoptotic cell death. To test whether the loss of pie function also causes similar defects in male GSCs, we analysed pie mutant clones. We observed that pie loss-of-function GSC clones could be detected 2 days after induction, but were rapidly lost 5 to 7 days after induction ( Supplementary Fig. 6b,d,f,h ). Control wild-type clones remained throughout these time points and were readily identified as GSCs, GBs and spermatogonia ( Supplementary Fig. 6 b,c,e,g ). Conversely, the overexpressing pie in the male germline under nos-Gal4 driver markedly increased male GSC population (vasa positive cells in direct contact with the somatic hub), compared with the nos-Gal4>GFP controls ( Supplementary Fig. 6l-n ). These data suggest a conserved role for pie in male GSC maintenance and proliferation. Pie is required for stem cell division To investigate the non-apoptotic role of pie in stem cells, we examined the pie mutant GSCs for division capacity. We compared the division rate of wild-type (GFP+, non-clonal) and mutant (GFP-, clonal) GSCs at 5 and 8 days after clonal induction. We found significantly reduced ‘division indices’ of pie GSCs compared to wild-type GSCs ( Fig. 3a-e , Supplementary Table 6 , Methods [25] ), indicating that pie is required for normal GSC cell division. Pie is required for cell division also in other stem cell types, since pie ISC clones in the midgut generate significantly fewer cells compared with the wild-type ISC clones ( Supplementary Fig. 7 ). Figure 3: pie is required for female GSC division. ( a ) Germarium of hsFlp; Ubi-GFP FRT40A/FRT40A females, 8 days after heat shock. ( b – c ) Germaria of hsFlp; Ubi-GFP FRT40A/ pie f05500 FRT40A females, 8 and 9 days after heat shock. ( d ) Germarium of hsFlp; Ubi-GFP FRT40A/ pie E1-16 FRT40A females, 8 days after heat shock. White arrow, clonal GSC; yellow arrow, non-clonal sister GSC; white dashed circle, progenies produced by clonal GSC within stage 1-2A. ( e ) Means of division indices of FRT40A , pie f05500 and pie E1-16 GSCs are calculated from samples collected, respectively, at 5 and 7-8 days after heat shock induction. Sample size specified in Supplementary Table 6 . Error, s.d. In ovaries 8 days after heat shock induction, pie f05500 clonal GSCs (white dashed circles and arrows) display repressed expression of Cyclin B ( f ), elevated expression of Cyclin E ( g ) and dacapo ( h ), compared with non-clonal sister GSCs (yellow dashed circles). ( i ) Means of frequencies of pie mutant ( pie f05500 and pie E1-16 ) GSCs positive for each cell cycle marker compared with those of non-clonal sister GSCs. Sample size specified in Supplementary Table 7 . Error, s.d. ( j ) Diagram of cell cycle phases and corresponding markers. Full size image To determine whether the division defects in stem cells are due to a block in the cell cycle progress, we analysed the distribution of cell cycle stages in pie mutant GSCs by staining mosaic germaria with antibodies against different cell cycle markers ( Fig. 3j ). We observed an increase of the frequencies of pie mutant GSCs staining positive for Cyclin A (CycA ), Cyclin E (CycE ) and Dacapo ( Dap ; a Drosophila homologue of the p21 ), and a decrease of GSCs positive for Cyclin B (CycB ), using two independent pie mutant alleles ( Fig. 3f-i , Supplementary Table 7 ). The frequencies of male GSCs with enhanced CycE level were also increased in both pie E1-16 and pie f05500 mosaic testes ( Supplementary Fig. 6I-k ). These data suggest a cell cycle defect in the pie mutant GSCs; possibly an arrest at the G1/S phase transition ( Fig. 3j ). Pie regulates stem cell self-renewal and division through FOXO Pie shares highly similar sequence with the PHD/RING domains of human G2E3 , an E3 ubiquitin ligase essential for mammalian early embryonic development. Biochemical evidence has demonstrated that these PHD/RING domains are responsible for the catalytic function of G2E3 (ref. 23 ). We show that the overexpression of His-pie in human 293T cells induces a marked ubiquitination in whole-cell lysate, confirming the role of pie as an E3 ligase ( Supplementary Fig. 8 ). The cell cycle profile of pie mutant GSCs described above shares high similarity with what have been reported for insulin receptor (InR)- deficient GSCs [25] , suggesting a potential connection between pie and InR signalling. As an E3 ligase that ubiquitinates protein for degradation, pie is likely to target a negative regulator in the InR signalling pathway. The primary candidate is FOXO , which is negatively regulated by InR signalling through the AKT- induced phosphorylation [26] . To test this hypothesis, we examined FOXO expression by immunostaining in pie mutant GSCs. Compared with neighbouring wild-type GSCs, pie mutant clonal GSCs display an upregulated level of FOXO protein in the nucleus ( Fig. 4a , marked by magenta dashed circle, quantified in Figure 4b , Supplementary Table 8 ). Importantly, the reduction of FOXO , using the foxo 25 /+ null allele in a heterozygous state, significantly rescued both the maintenance and the division phenotypes of pie mutant GSCs ( Fig. 4c-d ; Supplementary Table 9 ). These data conclusively indicate that pie promotes GSC self-renewal by repressing FOXO levels. In addition, we observed a significant increase of undifferentiated germ cells, marked by dotted fusomes, in the testes of foxo 21 /foxo 25 transheterozygotes compared to heterozygous controls ( Supplementary Fig. 9 ). We conclude that the reduction of FOXO is sufficient to promote GSC proliferation. Figure 4: pie regulates GSC self-renewal through FOXO level. ( a ) Eight to eleven days after clone induction, pie E1-16 clonal GSC nucleus (GFP−, magenta dashed circle) display higher expression of FOXO compared with sister non-clonal GSC nucleus (GFP+, white dashed circle). Yellow dashed circles mark the whole GSCs. ( b ) Quantification of relative FOXO expression levels (clonal versus non-clonal) in pie E1-16 GSCs and FRT40A controls. Sample sizes refer to Supplementary Table 8 . Error, s.d. ( c ) Heterozygous mutant foxo 25 /+ rescues the rapid loss of pie E1-16 GSCs. Each data point represents mean of three independent experiments. ( d ) Heterozygous mutant foxo 25 /+ rescues division defects of pie E1-16 GSCs. Sample sizes refer to Supplementary Table 9 . Error, s.d. ( e ) ISCs from wild-type midguts have undetectable FOXO level while pie RNAi knockdown ISCs stained positive for anti-FOXO antibody ( f , red arrows). Scale bar, 20 μm. ( g – h ) Posterior midguts of esgGal4, UAS-GFP>UAS-GFP ( g ) and esgGal4, UAS-GFP>UAS-FOXO ( h ) adults. Scale bar, 75 μm ( i ) Means of esgGFP+ cell numbers normalized to quantified gut area (esgGal4>GFP: n =15; esgGal4>FOXO: n =11). Error, s.d. ( j ) Eye disc from 3 rd instar larva with pie E1-16 clones (GFP-) and ( k ) fly eye developed into adulthood. ( l ) Eye disc from 3 rd instar larva with pie E1-16 ; foxo 25 /+ clones (GFP−) and ( m ) fly eye developed into adulthood. ( n ) Quantification of eye discs with or without apoptotic clones in pie E1-16 ( n =25) and pie E1-16 ; foxo 25 /+ ( n =22) larvae. Full size image Similarly, FOXO is undetectable in wild-type ISCs in the posterior midgut, but the depletion of pie through esgGal4 driven RNAi resulted in elevated FOXO protein levels specifically in the ISCs ( Fig. 4e-f , red arrows). Furthermore, the overexpression of FOXO in ISCs significantly reduced ISC population, phenocopying pie knockdown defects ( Fig. 4g-i ). These results indicate a conserved role for pie in regulating ISC proliferation by mediating FOXO level. FOXO is highly expressed in Drosophila larval fat bodies [27] . To investigate whether pie regulates FOXO at the level of RNA or protein, we examined FOXO expression after knocking down pie with fat body specific driver r4Gal4 (ref. 28 ). Compared with GFP controls ( Supplementary Fig. 10a ), knocking down pie markedly enhanced the FOXO protein level in the nuclei ( Supplementary Fig. 10b ). Conversely, the overexpression of pie in fat body cells display reduced FOXO protein levels ( Supplementary Fig. 10c ). Despite these changes in the protein level, neither the overexpression nor the knockdown of pie significantly affected FOXO mRNA levels, as quantified by quantitative PCR (qPCR) and normalized to internal control rp49 ( Supplementary Fig. 10d ). These data suggest that FOXO is regulated by pie at a post-transcriptional level. The cell survival role of pie in somatic tissue is through FOXO With the knowledge that pie has a self-renewal role in stem cells but an anti-apoptotic role in somatic cells, the next question is whether pie functions through the same pathway in both cell types. Pie mutant clones in 3 rd larval instar eye discs display high level of apoptosis marker, cleaved caspase 3 (ref. 24 ; Fig. 2c ; Fig. 4j ). The resulting adult eyes include very few mutant clones (white; Fig. 4k ). Strikingly, reducing FOXO level by introducing the heterozygous null mutation foxo 25 /+ in pie mutant background significantly rescued the apoptosis phenotype as indicated by diminished cleaved caspase 3 in eye discs ( Fig. 4l,n ). FOXO heterozygosity also rescued the pie mutant clones in the adult eyes ( Fig. 4m ). These results suggest that pie also regulates FOXO in somatic tissues, but the outcome of this regulation is repression of apoptosis. Drosophila pro-apoptotic protein, Hid (Head involution defective), Grim, Reaper and Sickle are collectively known as RHG proteins and repress the apoptosis inhibitor DIAP , thereby resulting in caspase activation and apoptosis. Drosophila RHG proteins are homologues of mammalian Smac/DIABLO proteins that function through binding and lowering the level of IAP [3] , [29] . Previous studies showed that DNA damage-induced apoptotic response in larval eye tissue is mediated by JNK/FOXO signalling, in which FOXO and Fos transcriptionally activate Hid [30] . To investigate whether Hid is also activated in pie mutant clones that undergo FOXO-dependent apoptosis, we examined Hid levels by immunostaining. In 3 rd instar eye discs, we observed a marked Hid expression in the pie−/− clones, co-localizing with activated caspase ( Supplementary Fig. 11 ). Tie-bantam- regulated Hid levels protect GSCs against apoptosis The data in the preceding sections show that loss of pie results in caspase activation and apoptosis in the larval eye discs and in differentiating EC cells of the midgut but not in stem cells. In agreement, while Hid was induced in pie mutant clones in the eye disc and in pie mutant cystoblasts ( Fig. 5a , yellow arrowhead, C, Supplementary Fig. 12 ), no increase in Hid expression was detected in pie mutant GSCs ( Fig. 5a , white arrow, C; Supplementary Table 10 ). This difference is particularly striking between the GSC and its daughter ( Fig. 5a ). The difference in Hid levels between pie stem cells and differentiating cells suggests an additional regulation on Hid specifically in the stem cells. Figure 5: Pvf1 from dying daughters activates Tie to protect stem cell from apoptosis through bantam-regulated hid level. ( a ) hsFlp;Ubi-GFP FRT40A/pie E1-16 FRT40A and ( b ) hsFlp;; armLacZ FRT80B/ banΔ1 FRT80B germarium 8 days after heat shock. Yellow dashed line circles clonal GSC and its CB daughter. White arrows: GSCs; yellow arrowheads: cystoblasts. ( c ) Means of percentage of hid+ clonal GSCs and non-clonal neighbor GSCs of pie E1-16 ( n =97) and banΔ1 ( n =57) background. NS: not significant. ( d ) Mean GSC numbers per germarium of w1118 ( n =44) and hs-Hid ( n =38) females, 1 day after heat shock treatment. ( e ) Means of percentage of germaria without GSCs in banΔ1/TM6 ( n =160) and hid l(3)05014 , banΔ1/TM6 ( n =191) females 3 days after IR. tie e03394 mutant germarium one day ( f ) and 3 days ( g – h ) post 50 Gy IR treatment. White dashed circles mark the somatic cap cells; yellow dashed circles indicate GSCs labelled by dotted spectrosomes (absent in h ); cleaved dcp-1 (green) indicates apoptotic cells. ( i ) Percentages of germaria with branched fusomes (green), with only GSCs (blue), and absent of any GSCs (red) are shown for w- ( n =204) and tie e03394 mutant ( n =270) 3 days post 50 Gy IR. ( j – l ) ban-GFP sensor activity quantified as intensity in GSCs (yellow dashed circles) normalized against follicle cells (green dashed outlined), in tie Df /+ ( n =12) and tie Df/Df ( n =8) females. ( m ) Percentages of germaria with branched fusomes (green), with only GSCs (blue), and absent of any GSCs (red) are shown for w- ( n =61), foxo 21 /+ ( n =105) and foxo 21 /foxo 25 mutants ( n =287) 3 days post IR. ( n ) w1118 germarium pre and ( o ) 1 day post 50 Gy IR. White dashed circles mark the cap cells; yellow dashed circles indicate GSCs labelled by dotted spectrosomes facing the niche; red dashed circles mark differentiated cystoblasts. Note Pvf1 expression is markedly elevated in the cystoblasts post IR ( o ). ( p ) Germarium of bamGal4/Pvf1 RNAi adults 3 days post 50 Gy IR. Apoptotic GSC shows cleaved dcp-1 activity (green). ( q ) Mean percentages of germaria absent of GSCs from various genotypes are shown. Sample size specified at the bottom. Note pvf1 MB01242 50 Gy d3 is highly significant (*** P ≤0.001) compared with either bamGal4/ +, 50 Gy d3 or pvf1 MB01242 50 Gy d0 . ( r ) Proposed mechanism of how female GSCs are protected against apoptosis through joint efforts from multiple signalling pathways. Error, s.d. Full size image Prior studies in imaginal discs showed that Drosophila microRNA bantam (ban) represses IR-induced apoptosis through targeting the 3′UTR of Hid (ref. 31 ). Our previous findings have demonstrated that ban is highly expressed in GSCs and required for GSC maintenance ( Supplementary Fig. 13 ) [32] . To test if ban also functions in stem cells by repressing Hid , we induced mutant clones of ban and stained for Hid . We observed a significant elevation of Hid expression in ban mutant GSCs, compared with the wild-type/heterozygous neighbours ( Fig. 5b-c , Supplementary Table 10 ). Strikingly, ban mutant GSCs show similar Hid level as their CB daughters ( Fig. 5b ). Forced expression of Hid , from a heat shock promoter, activates the downstream apoptotic pathway resulting in a rapid GSC loss one day after heat shock ( Fig. 5d , Supplementary Fig. 14 ). To test if ban-dependent repression of hid levels is required to protect GSCs from apoptosis, we examined banΔ1/TM6 and hid l(3)05014 , banΔ1/TM6 germaria 3 days post 50 Gy IR. While banΔ1 heterozygous mutant displayed severe GSC loss due to IR (52.25%), reduction of Hid level ( hid l(3)05014 , banΔ1/TM6 ) markedly rescued this phenotype (20.5%; Fig. 5e , Supplementary Fig. 15 ). These data reveal Bantam-dependent repression of Hid as a critical protection mechanism in GSC during genotoxic stress. The Hippo pathway is known to regulate ban in controlling cell proliferation and apoptosis [33] , [34] . However, ban does not appear to be regulated in this manner in the GSCs since yorkie mutant GSCs are maintained in the niche [32] , calling for a search of an independent pathway that regulates ban . Drosophila Tie , which encodes a receptor tyrosine kinase of VGFR/PDGFR family, has been identified as a dominant modifier of ban in IR-induced apoptosis [20] . In larval imaginal discs, Tie was found to be required for non-cell autonomous activation of ban in response to cell death, and the resulting ban activation prevents further IR-induced apoptosis [20] . Given the above-described evidence that ban normally acts to repress Hid in the GSCs, we tested if Tie also has a role in the resistance of GSCs against apoptosis. Homozygous tie mutant females are viable and fertile but following exposure to 50 Gy of IR, the germaria lost most germline cells including the GSCs ( Fig.5f-i , Supplementary Table 11 ). Caspase activation could be observed as early as one day after irradiation in the cystoblasts ( Fig. 5f ). Importantly, tie GSCs show caspase activation 3 days after irradiation ( Fig. 5g ), while caspase activation was rarely observed in irradiated wild-type controls ( Supplementary Fig. 16 ). Using a previously described ban-sensor [35] , we found that tie−/− GSCs exhibited elevated sensor signal, indicative of lower ban activity, compared with heterozygous controls ( Fig. 5j-l , Supplementary Table 12 ). On the basis on these results we conclude that Tie acts through ban to repress Hid levels and to protect GSCs from IR-induced apoptosis. It has been shown that three putative ligands for Tie , Pvf1, Pvf2 and CG10359 are induced upon IR in wing discs [36] . Genetics analysis shows that Pvf1 is required for the non-autonomous protective effect of dying cells, making it the most likely ligand for Tie in this context [20] . We analysed Pvf1 expression with immunostaining and noticed significantly elevated Pvf1 levels in the TA germ cells upon IR, especially in the cystoblasts ( Fig. 5n-o , red dashed circles), while GSCs exhibit undetectable Pvf1 expression, similar to nonirradiated germaria (yellow dashed circles). Examination of Pvf1-GFP enhancer trap germaria post IR show that Pvf1 is induced on transcriptional level in the TA germ cells after irradiation ( Supplementary Fig. 17 ). To further validate the source of the functional ligand that activates Tie in GSCs, we knocked down Pvf1 specifically in the neighbouring differentiating TA germ cells (cystoblasts and 2–8 cell cysts using bamGal4 driver [37] ), which is confirmed by the repressed Pvf1 expression on IR ( Supplementary Fig. 18 ). The GSCs adjacent to Pvf1 knockdown cysts became significantly sensitive to IR-induced apoptosis; 30% of the germaria lost GSCs completely after 3 days and the remaining GSCs in the niche show caspase activity ( Fig. 5p-q ; Supplementary Table 13 ). Similar effect was also detected in pvf1 MB0124 2 GSCs, but not observed in the absence of IR. In contrast, Pvf1 knockdown with c587Gal4 driver, which drives expression in most somatic cells throughout female gonad development [38] , did not sensitize GSCs to IR treatment, ruling out the somatic niche cells as potential source for the Pvf1 survival signal ( Fig. 5q ). To test whether FOXO and Tie pathway both act in GSC survival, or whether Tie is sufficient for the process, we tested the FOXO mutant stem cell survival capacity after IR. Importantly, FOXO mutant stem cells show significant loss after IR, suggesting that the correct FOXO levels are critical for stem cell survival ( Fig. 5m ). In this study we show that an anti-apoptotic gene, pie , is required for stem cell self-renewal but not for resistance to apoptosis, indicating a compensatory anti-apoptotic mechanism in stem cells. The cell cycle marker profile of pie GSCs resembles that of InR deficient GSCs, leading to our finding that pie controls GSC, as well as ISC self-renewal/division through FOXO protein levels. Surprisingly, pie targets FOXO as well in differentiating cells, failing to explain why the loss of pie does not induce apoptosis in stem cells. However, while the upregulation of FOXO leads to the upregulation of its apoptotic target Hid in differentiating cells, in adult stem cells Hid is not upregulated. Hence additional regulatory pathway is in place to repress Hid and thereby apoptosis in stem cells. We identified Tie-receptor as the key gatekeeper for the process in the GSCs. The signal ( Pvf1 ) from the dying daughter cells activates Tie in GSCs to upregulate bantam microRNA that represses Hid , thereby protecting the stem cells. Bantam is known to repress apoptosis and activate the cell cycle. However, while protected from apoptosis in this manner, the stem cells do not activate the cell cycle but rather stay in protective quiescence through FOXO activity ( Fig. 5r ). When the challenge is passed, stem cells repopulate the tissue. The mammalian pie homologue, G2E3 was reported to be an ubiquitin ligase with amino terminal catalytic PHD/RING domains. G2E3 is essential for early embryonic development [23] . Importantly, microarray data show significant enrichment of G2E3 expression levels in human embryonic stem (ES) cell lines [39] . These observations suggest a critical role of G2E3 in embryonic development, potentially in maintaining the pluripotent capacity. Since FOXO is shown to be an important ESC regulator [40] , [41] , it will be interesting to test whether defects in G2E3 result in changes in FOXO levels. Furthermore, future studies are required to test whether human ES cells also are protected from apoptosis due to external signals from dying neighbouring cells ( Fig.5r ). The cell cycle defects of pie mutant stem cells, such as abnormal cell cycle marker profile, can be a consequence of elevated FOXO levels, since FOXO is a transcription factor with wide array of target genes, many of which are involved with cell cycle progress, such as the cyclin-dependent kinase inhibitor p21/p27 ( Dacapo in Drosophila ) [42] . This may be critical when bantam function is considered in the stem cells. Bantam is known to function as anti-apoptotic and cell cycle inducing microRNA [31] , [33] , [34] . While in GSC bantam is critical through its anti-apoptotic function as a Hid repressor, it has no capacity to induce GSC cell cycle after irradiation. In a challenging situation, such as irradiation, an additional protection mechanism for the tissue is to keep the stem cell in a quiescent state during challenge. bantam’s pro-cell division activity may be dampened by FOXO’s capacity to upregulate p21/Dacapo . The FOXO family is involved in diverse cellular processes such as tumor suppression, stress response and metabolism. The FOXO group of human Forkhead proteins contains four members: FOXO1, FOXO3a , FOXO4 , and FOXO6 . Studies to elucidate their function in various stem cell types in vivo using knockout mice have shown some potential redundancy of FOXO proteins. Recent publications have demonstrated a requirement for some of the FOXO family members in mouse hematopoietic stem cell proliferation [43] , mouse neural stem cells [44] , leukaemia stem cells [45] and human and mouse ES cells in vitro [41] . However, FOXO is shown to be dispensable in the early embryonic development in mouse [46] . Drosophila genome has only one FOXO , allowing a definitive study of FOXO’s function in stem cells. We now demonstrated that tight regulation of FOXO protein levels is essential for in vivo GSC and ISC self-renewal in Drosophila . While the loss of FOXO function generates supernumerary stem cells, inappropriately high level of FOXO results in stem cell loss. Under challenge, such as exposure to irradiation, stem cells depleted of FOXO fail to stay quiescent and become more sensitive to the damage, leading to the loss of GSC population ( Fig. 5m ). These data demonstrate the importance of the balanced FOXO expression level for stem cell fate. Previous studies have shown that multiple adult stem cell types manage to avoid cell death in response to severe DNA damage [47] . We studied the mechanisms that stem cells utilize to avoid apoptosis in absence of pie and revealed that apoptosis is protected through a receptor, Tie and its target miRNA bantam that can repress the pro-apoptotic gene Hid . We show that the ligand for Tie is likely secreted from the dying neighbours since Tie is essential in GSC only after irradiation challenge, IR induces Tie 's potential ligand Pvf1 expression in cystoblasts and knockdown of Pvf1 in cystoblasts eliminates stem cells’ protection against apoptosis. Further studies will reveal whether the same protective pathway is utilized in other stem cells. Community phenomenon have been described previously around dying cells: compensatory proliferation, Phoenix rising, bystander effect and Mahakali [20] , [48] , [49] , [50] . While Bystander effect describes dying cells inducing death in the neighbours, compensatory proliferation, Phoenix rising and Mahakali describe positive effects in cells neighbouring the dying cells [20] , [48] . The present work shows that adult stem cell can survive but show no immediate induction of proliferation when neighboured by dying cells. However, since adult stem cells can repopulate the tissue when death signals have passed, we propose that in adult stem cells these phenomenon merge. First, the GSCs survive by bantam repressing the apoptotic inducer, Hid , and later repopulate the tissue by activating cell cycle. Recent findings have suggested that p53 might play an important role in re-entry to cell cycle in stem cells [51] . The results from our studies shed light on the general understanding of stem cell behaviour in response to surrounding tissue to ensure the normal tissue homeostasis. It is also plausible that cancer stem cells hijack these normal capacities of stem cells. Fly stocks and culture conditions The following stocks are obtained from the Bloomington Drosophila Stock Center at Indiana University: pie 54 /SM1, pie EB3 /CyO, yw, hsFLP;Ubi-GFP FRT40A/CyO, w; FRT40A/CyO, hsFLP;FRT42BUbi-GFP/CyO, w; UAS-GFP/CyO, nanos-Gal4 (NGT40; nanos-Gal4:VP16), yw;; r4Gal4, Df(3L)Exel9028, PBac{RB5.WH5}Exel9028 (Tie Df ), Pvf1 RNAi (y1 sc* v1; P{TRiP.HMS01958}attP40 and Pvf1 enhancer trap Mi{ET1}Pvf1 MB01242 . RNAi stocks, pie RNAi (22094) and pie RNAi (22095)/CyO are from Vienna Drosophila RNAi Center (VDRC). yw; pie f05500 P{neoFRT}40A/CyO was obtained from the Drosophila Genetic Resource Center, the Kyoto Institute of Technology, Japan. w; pie E1-16 FRT40A/SM5-TM6B was a generous gift from Nicholas E. Baker. esg-Gal4, UAS-GFP/ CyO from Bruce Edgar; foxo 21 and foxo 25 from Ernst Hafen; UASp-FOXO from Linda Partridge; w; myoIAGal4/CyO; tubGal80ts UAS-GFP/TM6B and UAS-GFP flp122; FRT40A tubGal80; tubGal4/TM6B from Jin Jiang; w;; diap1 22-8s FRT80B and amorphic allele hid l(3)05014 from Hermann Steller; w;Su(H)GBE-Gal4 UAS-GFP/CyO from Steve Hou; w; p[GBE + Su(H) m8, ry+, lacZ] from Craig Micchelli; w - ;;Df(3L)banΔ1 FRT80B/TM6 (ref. 35 ), pBAC{RB}Tie e03394 (Harvard Exelixis Collection); bamGal4 from Ting Xie; c587Gal4 from Cai Yu and hs-Hid from Matt Mahoney. Flies were cultured at 25 °C on standard cornmeal-yeast-agar medium unless stated otherwise. Gamma-irradiation and maytansinol treatment Young adult flies with specific phenotype are collected (<5 days old) and transferred into empty vials without food. Irradiation is applied with Cs-137 Mark I Irradiator according to instructed dosage chart. Post-treatment animals are transferred back to fresh food and maintained at room temperature until desired time points. Maytansinol is diluted in serial concentrations in grape juice and given to young flies on filter paper every day. Immunofluorescence and microscopy Adult ovaries, testes, midguts or fat bodies from 3 rd instar larvae of desired genotypes were dissected in PBS and immediately fixed in PBS containing 4% paraformaldehyde. Samples are then washed with PBT (PBS containing 0.2% Triton X-100), blocked in PBTB (PBT containing 0.2% BSA, 5% normal goat serum) and incubated with primary antibodies overnight [52] . The following primary antibodies were used: mouse anti-adducin, mouse anti-Lamin C, mouse anti-FasIII, mouse anti-Cyclin A, mouse anti-Cyclin B, mouse anti-delta (Developmental Studies Hybridoma Bank, 1:20), rabbit anti-cleaved caspase 3 (Cell Signaling Technology, 1:250), rabbit anti-cleaved Drosophila dcp-1 (Cell Signaling Technology, 1:250), rabbit anti-phospho-Histone3 (Upstate Biotechnology, 1:250), rabbit anti-Cyclin E (Santa Cruz Biotech, 1:50), rabbit anti-FOXO (generous gift from Pierre Léopold, 1:500), anti-Vasa (gift from P. Lasko, 1:1,000), mouse anti-dacapo (NP1, gift from Mary Lilly, 1:10), guinea pig anti-Hid (1:100, gift from Hyung Don Ryoo), rat anti-Pvf1 (gift from Ben-Zion Shilo, 1:100), rabbit anti-GFP (Molecular Probes, 1:2,000) and rabbit anti-βGal (1:5,000). After washes with PBT, secondary fluorescence antibodies were utilized including Alexa 488, 568, 633 anti-mouse, anti-rabbit, anti-rat and anti-guinea pig (1:250). The samples were mounted and analysed on Leica SPE5 and Nikon N1 confocal laser-scanning microscopes. Images are representative of >3 experiments unless stated otherwise. Generation of clones Clones of GSCs were induced using the heat shock FLP-FRT system [53] , [54] . Females or males (2–4 days old) of the following genotypes hsFLP;Ubi-GFP FRT40A/GFP FRT40A, hsFLP; Ubi-GFP FRT40A/ pie E1-16 FRT40A, hsFLP;Ubi-GFP FRT40A/pie f05500 P{neoFRT}40A were heat shocked for 45 min in 37 °C water bath for two consequent days to induce mitotic recombination. hsFlp;; armLacZ FRT80B/ bantamΔ1 FRT80B and hsFlp;; ubi-GFP FRT80B/diap1 22-8s FRT80B adult females were heat shocked for 2 × 30 min in 37 °C water bath for two consequent days. Heat shocked flies were kept at 25 °C and transferred to fresh food with wet yeast paste every other day before dissection. MARCM clones in midgut were generated as previously described [55] : fly stocks were crossed to generate the following genotypes: UAS-GFP flp122; tubGal80 FRT40A /FRT40A; tubGal4/+, UAS-GFP flp122; tubGal80 FRT40A / pie E1-16 FRT40A; tubGal4/+, UAS-GFP flp122; tubGal80 FRT40A/pie f05500 FRT40A; tubGal4/+. To induce MARCM clones, female flies were heat shocked in a 37 °C water bath for 45 min and kept at 29 °C afterwards until desired time points. Division index analysis Only germaria containing both GFP-positive and GFP-negative GSCs were analysed for cell division. The average sum of cystoblasts and cysts generated by individual GFP-negative GSCs in region 1-2A of a germarium was normalized to that of individual GFP-positive control heterozygous GSCs to obtain the division index [25] , [56] . Generation of pUASp-pie plasmid and transgenic lines The pie insert was generated by PCR from the Berkeley Drosophila Genome Project cDNA library using 5′-GGAGGTACCATGGAAGATAACAAGGAGCTGCAATGCTTAA-3′ and 5′-GCCTCTAGATTAAGAGAACCCCTCTGATCTGTACCATTCGTGG-3′ primers, and cloned into the KpnI and XbaI sites of the pUASP vector [57] . Transgenic flies were generated by injection of purified plasmid DNA into w1118 Drosophila embryos (Rainbow Transgenic Flies, Newbury Park, CA, USA). These flies were crossed with w1118 and transformants were selected based on eye colour. Quantitative real-time PCR Third instar larvae of desired genotype were dissected in PBS and fat bodies were collected and washed with PBS. Total RNA was isolated using Trizol (Invitrogen) according to the manufacture’s instruction. The cDNA was generated from purified RNA using Omniscript RT kit (QIAGEN). The cDNA was then used as template for qPCR analysis using SYBR green-based detection on a BioRad iCycler. Results were quantified using the delta–delta Ct method to normalize to rp49 transcript levels and to the control genotypes. Data presented are averages and s.d. from at least three independent biological repeats. The following primer pairs were used. Rp49: 5′-AATCTCCTTGCGCTTCTTGGAGGA-3′, 5′-AAGAAGTTCCTGGTGCACAACGTG-3′ Pie: 5′-GCAAATGCGTTGAGAGTAGC-3′, 5′-TGGAAGATAACAAGGAGCTGC-3′ FOXO: 5′-GAGTCAGATTTACGAGTGGATGG-3′, 5′-TTTGGACCCTCATAAAGCGG-3′. Cell transfection and western blot Human HEK293FT cells (Invitrogen) are transfected with Lipofectamine 2000 (Invitrogen) for 48 h following instruction. Cells are lysed on culture dish and followed with western blot assay [58] . Protein concentration was determined by BCA protein assay system (Thermo Scientific, Rockford, IL). Antibodies used include: anti-his HRP conjugated antibody (Qiagen, 1:10000); anti-ubiquitin antibody (Santa Cruz Biotech, 1:10,000); β-actin antibody (Santa Cruz Biotechnology, 1:10,000). In brief, cells were washed with DPBS and directly lysed on culture dish using homogenizing buffer consisting of 20 m M Tris-HCl (pH 7.5), 150 m M NaCl, 15% Glycerol, 1% Triton, 3% SDS, 25 m M β-glycerolphosphate, 50 m M NaF, 10 m M NaPyrophosphate, 0.5% Orthovanadate, 1% PMSF (all chemicals are from Sigma-Aldrich, St Louis, MO), 25 UBenzonase Nuclease (EMD Chemicals, Gibbstown, NJ) and protease inhibitor cocktail (Complete Mini, Roche Applied Science, Germany). Protein extracts (20 μg) were loaded, separated by 7.5% SDS–PAGE, and transferred to polyvinylidene difluoride membranes (Hybond-N+, Amersham Pharmacia Biotech, Buckinghamshire, England). Membranes were blocked with 5% nonfat dry milk for at least 60 min at room temperature, and incubated overnight at 4 °C with primary antibody. Finally, after the blots had been incubated for 1 h with horseradish peroxidase-conjugated secondary antibodies, they were visualized by enhanced chemiluminescence (Millipore Corp, Billerica, MA). Quantification of ISCs For each midgut sample analysed, scans were taken from three spots on posterior midgut under the same magnification. Average ISC numbers were calculated by the total number of esgGFP positive cells from the three scans and normalized to the total area scanned. The area of each scan was analysed using ImageJ software. Statistical analysis Throughout the paper, statistical significance was calculated as P values using two-tailed Student's t -test. *, P ≤0.05; **, P ≤0.01; ***, P ≤0.001 and **** P ≤0.0001. Error bars show s.d. for at least three independent experiments. How to cite this article : Xing, Y. et al . Tie-mediated signal from apoptotic cells protects stem cells in Drosophila melanogaster. Nat. Commun. 6:7058 doi: 10.1038/ncomms8058 (2015).